Behavioural and neurobiological implications of linear and non-linear features in larynx phonations of horseshoe bats Mammalian vocalizations exhibit large variations in their spectrotemporal features, although it is still largely unknown which result from intrinsic biomechanical properties of the larynx and which are under direct neuromuscular control. Here we show that mere changes in laryngeal air flow yield several non-linear effects on sound production, in an isolated larynx preparation from horseshoe bats. Most notably, there are sudden jumps between two frequency bands used for either echolocation or communication in natural vocalizations. These jumps resemble changes in ‘registers’ as in yodelling. In contrast, simulated contractions of the main larynx muscle produce linear frequency changes, but are limited to echolocation or communication frequencies. Only by combining non-linear and linear properties can this larynx, therefore, produce sounds covering the entire frequency range of natural calls. This may give behavioural meaning to yodelling-like vocal behaviour and reshape our thinking about how the brain controls the multitude of spectral vocal features in mammals. Echolocating bats produce a wide variety of different sonar pulses and also have a rich repertoire of communication calls. In horseshoe bats, for example, a long constant frequency (CF) component characterizes their echolocation pulses. When the bat is perched (‘at rest’), it emits the CF portion of its echolocation calls at its so-called ‘resting frequency’ ( RF 2 ), which normally represents the second harmonic of the calls [1] . The pulses usually terminate with a brief and rapid drop in frequency and sometimes also contain an initial brief frequency rise, each extending 10–15 kHz below RF 2 . During flight, horseshoe bats change their CF frequency by up to 5 kHz below and 1–2 kHz above RF 2 [1] , [2] , [3] to compensate for Doppler shifts in the returning echo signal. This maintains the echo frequency practically constant (Doppler-shift compensation, DSC [1] ). Communication signals of horseshoe bats, on the other hand, are spectro-temporally more complex. Their second harmonic frequencies are more than 15 kHz below the RF 2 of echolocation pulses [4] . It is still unknown, however, how the bat larynx can produce such low call frequencies. In our present study, we chose a simplified approach as an initial step towards tackling the question of how the horseshoe bat larynx could generate the entire range of call frequencies observed in natural vocalizations. We used an isolated larynx preparation from these bats, which lacked any neuronal innervation, to test if we could reproduce the same range of frequencies in larynx phonations by merely changing the air flow in this preparation. If so, this would indicate that direct neuromuscular control by larynx muscles is not necessary. Instead, sound production would largely result from intrinsic biomechanical properties of the larynx. Alternatively, we examined if we could generate the same frequency range by simulating cricothyroid contractions in our larynx preparation. This directly addresses which role the neuromuscular control by the cricothyroid has in call frequency production. We found that changes in laryngeal air flow yielded several non-linear effects on sound production, most notably sudden jumps between two independent frequency bands, reminiscent of changes in ‘registers’, as in yodelling. These frequency bands matched the frequency ranges used for either echolocation or communication in natural vocalizations. On the other hand, simulated contractions of the main larynx muscle produced linear frequency changes, but only within each of the bands used for echolocation or communication. Therefore, only by combining non-linear and linear operational modes, that is, intrinsic properties and neuromuscular control, can the horseshoe bat larynx produce sounds covering the entire frequency range of natural calls. Frequencies for communication are lower than for echolocation In horseshoe bats, the second harmonic frequencies of communication calls are more than 15 kHz below the RF 2 of echolocation pulses [4] (vertical pairs of arrows in Fig. 1 ). Interestingly, neurophysiological recordings of the spike activity [5] in various motor structures demonstrate that their activity virtually ceases at call frequencies only 4–6 kHz below RF 2 . These structures include the cricothyroid muscle, which is the sole laryngeal muscle controlling call frequencies in bats [6] , its motor nerve, the superior laryngeal nerve [7] , and neurons within the motor nucleus of laryngeal control, the nucleus ambiguus itself ( Fig.2 ; surgery and stereotaxic approaches follow those outlined in detail in [8] , and the behavioural tests resulting in call frequency changes are identical to those published previously [9] , [10] ). Although this frequency range is sufficient to account for call frequencies produced during DSC, it poses a challenge for explaining how such extremely low-discharge patterns can encode for the low frequencies and large spectral modulations seen in communication calls. In addition to direct tension control of the mammalian vocal fold by a single larynx muscle, however, other mechanisms may also exist that affect tension and thus sound frequency [11] , [12] , [13] , [14] , [15] . 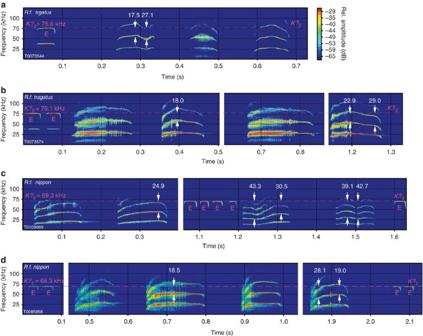Figure 1: Sonagrams of typical echolocation and communication calls from two subspecies of greater horseshoe bats. R. f. tragatus(two individuals inaandb, respectively) andR. f. nippon(two individuals incandd, respectively). Individual resting frequencies (RF2) of echolocation pulses (marked by ‘E’) given for each bat and indicated by pink hatched lines. Note the large frequency differences betweenRF2and the second harmonic of communication calls, which are indicated as numbers (kHz) above the white vertical pairs of arrows. Figure 1: Sonagrams of typical echolocation and communication calls from two subspecies of greater horseshoe bats. R. f. tragatus (two individuals in a and b , respectively) and R. f. nippon (two individuals in c and d , respectively). Individual resting frequencies ( RF 2 ) of echolocation pulses (marked by ‘E’) given for each bat and indicated by pink hatched lines. Note the large frequency differences between RF 2 and the second harmonic of communication calls, which are indicated as numbers (kHz) above the white vertical pairs of arrows. 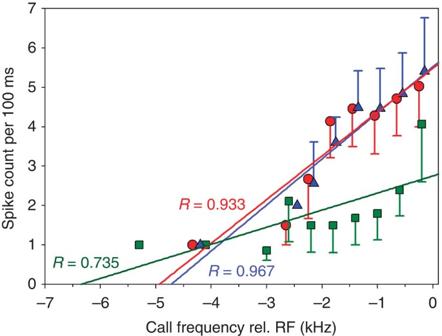Figure 2: Changes in spike activity with echolocation call frequency in laryngeal motor neurons. Spike activity virtually ceases in three single neurons in the laryngeal motor nucleus, the nucleus ambiguus. Data points represent means (bin width: 0.4 kHz)±s.d. (error bars). Outliers for low call frequencies are given without error bars. Rel., relative. Full size image Figure 2: Changes in spike activity with echolocation call frequency in laryngeal motor neurons. Spike activity virtually ceases in three single neurons in the laryngeal motor nucleus, the nucleus ambiguus. Data points represent means (bin width: 0.4 kHz)±s.d. (error bars). Outliers for low call frequencies are given without error bars. Rel., relative. Full size image Testing sound production in isolated horseshoe bat larynges To determine how horseshoe bat larynges may be able to generate the entire frequency range of echolocation and communication call frequencies, we excised larynges from 11 greater horseshoe bats, Rhinolophus ferrumequinum (five males, six females) post mortem to produce an in vitro model of vocalization by varying tracheal air pressure. Adapting the approach by Fee et al . [16] for the bird syrinx, we removed larynx, trachea and both lung lobes from the bat, cleaned them of excess connective tissue and mounted them on the experimental platform. The vocal tract was cut immediately dorsal to the epiglottis ( Fig. 3a , Methods). 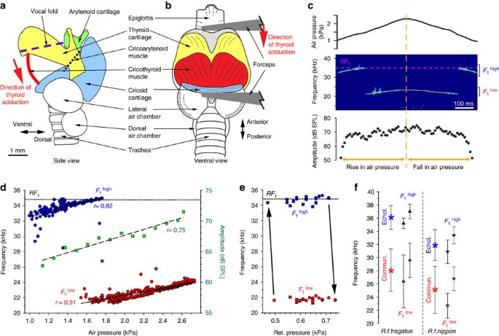Figure 3: Linear and non-linear frequency changes caused by varying air pressure. Side (a) and ventral view (b) of excised larynx. Instead of using direct action of a vocalis muscle to change vocal fold tension, echolocating bats tilt the thyroid cartilage through action of the cricothyroid muscle (a) in a visor-like fashion. This tautens the vocal folds, resulting in higher frequencies. Direction of thyroid adduction towards cricoid, simulating cricothyroid contraction, indicated by red arrow (a,b). (c–e) Sounds generated by excised larynx (Bat 1,Table 1) during slow changes in air flow. Frequency increases linearly for rising air pressures until it suddenly jumps from higher (F1high) to lower (F1low) frequencies. All frequency changes reverse for decreasing air pressures.F1highcorresponds to echolocation (Echol.) andF1lowto communication (Commun.) call frequencies. (c) Subglottal air pressures (top), sound fundamental frequency (F1; centre) and amplitude (bottom). Dashed line in centre trace: ‘resting frequency’,RF1, determined in live animal. (d) Variations in subglottal air pressure and changes in sound frequency (blue and red dots) and amplitude (green squares). Same preparation asc(ten increases and decreases of air pressure, each). Rate of linear changes in frequency forF1high(blue dots): 2.94 kHz kPa−1, andF1low(red dots): 2.4 kHz kPa−1. Horizontal dashed line andRF1: fundamental component of RF of this animal determinedin vivo. (e) Hysteresis of sudden, non-linear changes in sound frequency. Same data asd. Arrows: upper and lower ranges of sudden frequency shifts during increases (blue and red dots) and decreases (red and blue squares) of air flow, respectively. (f) Mean (symbols) and s.d. (error bars) ofF1high(blue triangles) andF1low(red triangles) produced by two larynx preparations forR. f. tragatus(left) andR. f. nippon(right). Ten trials each for increasing and decreasing air pressure. Asterisks: means of fundamental frequencies of Echol. (blue asterisks) and Commun. calls (red asterisks).R. f. tragatus:RF134.5–39.2 kHz (n=32 bats, mean: 36.1±1.82 kHz) and Commun. calls: 20.4–39.1 kHz (n=32 bats; mean: 28.1±3.23 kHz).RF1inR. f. nippon: 29.7–34.9 kHz (n=25 bats, mean 31.9±2.33 kHz) and Commun. calls: 14.4–33.4 kHz (n=25 bats; mean: 25.1±3.58 kHz). Rel., relative. Figure 3: Linear and non-linear frequency changes caused by varying air pressure. Side ( a ) and ventral view ( b ) of excised larynx. Instead of using direct action of a vocalis muscle to change vocal fold tension, echolocating bats tilt the thyroid cartilage through action of the cricothyroid muscle ( a ) in a visor-like fashion. This tautens the vocal folds, resulting in higher frequencies. Direction of thyroid adduction towards cricoid, simulating cricothyroid contraction, indicated by red arrow ( a , b ). ( c – e ) Sounds generated by excised larynx (Bat 1, Table 1 ) during slow changes in air flow. Frequency increases linearly for rising air pressures until it suddenly jumps from higher ( F 1 high ) to lower ( F 1 low ) frequencies. All frequency changes reverse for decreasing air pressures. F 1 high corresponds to echolocation (Echol.) and F 1 low to communication (Commun.) call frequencies. ( c ) Subglottal air pressures (top), sound fundamental frequency ( F 1 ; centre) and amplitude (bottom). Dashed line in centre trace: ‘resting frequency’, RF 1 , determined in live animal. ( d ) Variations in subglottal air pressure and changes in sound frequency (blue and red dots) and amplitude (green squares). Same preparation as c (ten increases and decreases of air pressure, each). Rate of linear changes in frequency for F 1 high (blue dots): 2.94 kHz kPa −1 , and F 1 low (red dots): 2.4 kHz kPa −1 . Horizontal dashed line and RF 1 : fundamental component of RF of this animal determined in vivo . ( e ) Hysteresis of sudden, non-linear changes in sound frequency. Same data as d . Arrows: upper and lower ranges of sudden frequency shifts during increases (blue and red dots) and decreases (red and blue squares) of air flow, respectively. ( f ) Mean (symbols) and s.d. (error bars) of F 1 high (blue triangles) and F 1 low (red triangles) produced by two larynx preparations for R. f. tragatus (left) and R. f. nippon (right). Ten trials each for increasing and decreasing air pressure. Asterisks: means of fundamental frequencies of Echol. (blue asterisks) and Commun. calls (red asterisks). R. f. tragatus : RF 1 34.5–39.2 kHz ( n =32 bats, mean: 36.1±1.82 kHz) and Commun. calls: 20.4–39.1 kHz ( n =32 bats; mean: 28.1±3.23 kHz). RF 1 in R. f. nippon : 29.7–34.9 kHz ( n =25 bats, mean 31.9±2.33 kHz) and Commun. calls: 14.4–33.4 kHz ( n =25 bats; mean: 25.1±3.58 kHz). Rel., relative. Full size image All 11 excised larynges exhibited consistent phonations to repeated trials of changes in subglottal air pressure. Because of the large number of experimental parameters that we tested and variations in the surgical extraction of larynges, we were not able to test all parameters in all preparations. The results of each of our experimental manipulations are based on at least two preparations (actual numbers given below). All sounds had their dominant frequencies at the fundamental ( F 1 ), because the excised larynx preparation lacked the resonance cavities (especially of pharynx and nose) that, in the vocal tract of live horseshoe bats, shift the peak frequencies towards the second harmonic of the naturally produced calls [17] , [18] , [19] . The range of absolute air pressures that we used to elicit phonations in the excised larynges varied between 1.5 and 3 kPa. It was thus well within the normal range of subglottal air pressures measured in naturally vocalizing bats (0.9–5.9 kPa) (ref. 20 ). The sound amplitudes for F 1 ranged from 63 to 82 dB SPL (median: 70.2±7.43 dB SPL). The second harmonic was on average 23.8±7.40 dB weaker. Changing air pressure We were able to test the effects of increases and decreases of air pressure on the production of tonal sounds in a total of six preparations. Figures 3 and 4 depict typical results. At the lowest subglottal air pressures that phonated the excised larynx (at approximately 1.1 kPa), the sounds had fundamental frequencies between 30 and 40 kHz ( F 1 high ; Fig. 3c-f ). This corresponded to the range of the fundamental in naturally produced echolocation calls. The lowest air pressures produced the lowest sound frequencies, which were always more than 2 kHz below the bat’s resting fundamental frequency ( RF 1 ; Fig. 3c ). Further increases in air pressure yielded a slow gradual rise in F 1 high (Pearson’s correlation, P <0.001, n =17) over an average range of 2.76±0.67 kHz, until a sudden and rapid drop of 13.1±0.03 kHz occurred that resulted in a lower F 1 ( F 1 low ). This F 1 low was unrelated with F 1 high ( Table 1 ). The sudden jump in sound frequency occurred within a pressure change of less than 0.05 kPa ( Fig. 3d ; Supplementary Fig. S1 ). Further increases in laryngeal air flow restored the smooth, graded rise in sound frequency (Pearson’s correlation, P <0.001, n =17) over an average range of 3.25±0.81 kHz, though at a lower fundamental frequency ( Fig. 3c ). The rates of frequency change in the other five preparations tested were similar and there was no significant difference for changes of F 1 high and F 1 low between preparations (paired t -tests, P >0.05, n =51). 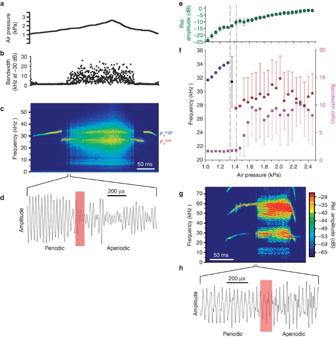Figure 4: High air pressures cause aperiodic larynx phonations. Below 2.1 kPa, changes are similar to those shown inFig. 3. Above 2.1 kPa, the tonal (periodic) signal suddenly becomes aperiodic. Similar aperiodic components are also part of natural communication (Commun.) calls. (a) Increases in air pressure, (b) bandwidth of sound signal 30 dB below max sound amplitude, (c) sonogram of produced sound and (d) waveform of sound signal for sudden transition between periodic and aperiodic sound emission (red box). (e,f) Effects of changes in absolute air pressure on relative amplitude (e), as well as sound frequency (f, left ordinate and blue and red dots) and signal bandwidth (f, bottom, right ordinate and pink squares). Same larynx preparation as in (a–d). Data represent averages of ten increases and decreases of air pressure, each. Vertical bars ine,frepresent s.d. and vertical dashed lines indicate the range of air pressure for rapid shifts betweenF1highandF1low. (g,h) Transition between periodic and aperiodic components in sonagram (g) and waveform (h, red box) of natural communication call ofR. f. nippon. Rel., relative. Figure 4: High air pressures cause aperiodic larynx phonations. Below 2.1 kPa, changes are similar to those shown in Fig. 3 . Above 2.1 kPa, the tonal (periodic) signal suddenly becomes aperiodic. Similar aperiodic components are also part of natural communication (Commun.) calls. ( a ) Increases in air pressure, ( b ) bandwidth of sound signal 30 dB below max sound amplitude, ( c ) sonogram of produced sound and ( d ) waveform of sound signal for sudden transition between periodic and aperiodic sound emission (red box). ( e , f ) Effects of changes in absolute air pressure on relative amplitude ( e ), as well as sound frequency ( f , left ordinate and blue and red dots) and signal bandwidth ( f , bottom, right ordinate and pink squares). Same larynx preparation as in ( a – d ). Data represent averages of ten increases and decreases of air pressure, each. Vertical bars in e , f represent s.d. and vertical dashed lines indicate the range of air pressure for rapid shifts between F 1 high and F 1 low . ( g , h ) Transition between periodic and aperiodic components in sonagram ( g ) and waveform ( h , red box) of natural communication call of R. f. nippon . Rel., relative. Full size image Table 1 Frequency profiles for individual bats. Full size table All frequency shifts, slow-graded as well as non-linear sudden jumps, reversed for decreases in air pressure ( Fig. 3c-e ). Slow decreases in F 1 high as well as F 1 low for decreasing air pressures occurred at the same rate as the rises in frequency for increasing air flows (no significant difference; paired t -test, P >0.05, n =17). The amount of frequency drop or rise that occurred during sudden, non-linear changes did not differ between increases and decreases of air pressure ( Table 1 ; paired t -test, P >0.3, n =51). However, the absolute frequency values at which the sudden changes took place did differ; for increasing air pressures, the sudden drops occurred at significantly higher pressures and, therefore, higher frequencies than the sudden rises during decreases in air flow ( Fig. 3e , paired t -test, P <0.001, n =17). The frequency values for the jumps were very consistent in each preparation, resulting in a very robust hysteresis behaviour. Interestingly, sudden non-linear jumps in frequency were not accompanied by sudden shifts in sound amplitude. Instead, sound amplitude continued to rise (or fall) linearly with further increases (or decreases) in subglottal air pressure ( Figs 3c and 4b ; R =0.75, Pearson’s correlation, P <0.001, n =17). Were the values of F 1 high and F 1 low related to any naturally produced call frequencies? We found that F 1 high matched the frequency range of the fundamental CF component of echolocation calls emitted at rest ( RF 1 ), whereas F 1 low overlapped with the range of fundamental frequencies in communication calls for individuals of Rhinolophus ferrumequinum tragatus in our colony of captive horseshoe bats [4] ( Fig. 3f left; paired t -test, P >0.3, n =23). Interestingly, we found that such a match also occurred in another subspecies of horseshoe bats, Rhinolophus ferrumequinum nippon , which generally emitted lower call frequencies ( Fig. 3f , right; paired t -test, P >0.3, n =16). When we increased subglottal air pressure to even higher levels than the maximum levels depicted in Figs 3 , 6 preparations, we observed yet another non-linear effect in addition to the sudden drop from F 1 high to F 1 low described above. Sound production suddenly switched from periodic (tonal) signals at F 1 low to aperiodic (chaotic) emission of signals. These aperiodic signals had bandwidths of more than 10 kHz mainly around F 1 low ( Fig. 4 ). The switch from periodic to aperiodic sounds occurred within less than 200 μs or only two to three cycles of the tonal signal. Decreasing the air pressure reversed the effect, and the signal switched back to a tonal sound emitted at F 1 low . Figure 6: Effects of simulated cricothyroid contractions on phonation frequencies. 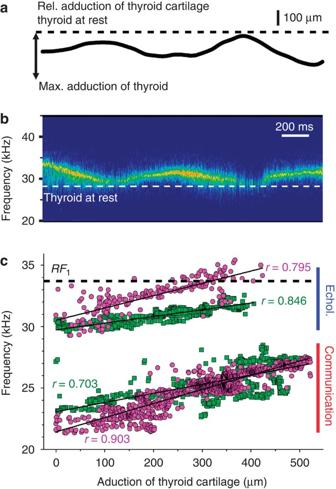Figure 6: Effects of simulated cricothyroid contractions on phonation frequencies. Different degrees of adduction of the thyroid (simulated contraction of cricothyroid muscle) on sound frequency caused frequency changes that were highly linear but limited to sounds emitted either withinF1highor F1low. (a) Different degrees of adduction of the thyroid towards the cricoid cartilage (top panel), and (b) resulting changes in sound frequency. Air pressure was maintained constant at a level yielding sounds emitted atF1high. (c) Frequency changes for two preparations (pink dots and green squares, respectively; both fromR. f. nippon) caused by adduction of the thyroid over a distance up to ~500 μm towards the cricoid cartilage (ten trials each). Pink dots depict same preparation as shown inaandb, and horizontal dashed line indicates the fundamental of the resting frequency (RF1=34.8 kHz) for this animal obtainedin vivo. Ranges of echolocation (Echol.)pulses and communication calls for this subspecies indicated at right (same data as inFig. 3f). Different degrees of adduction of the thyroid (simulated contraction of cricothyroid muscle) on sound frequency caused frequency changes that were highly linear but limited to sounds emitted either within F 1 high or F 1 low . ( a ) Different degrees of adduction of the thyroid towards the cricoid cartilage (top panel), and ( b ) resulting changes in sound frequency. Air pressure was maintained constant at a level yielding sounds emitted at F 1 high . ( c ) Frequency changes for two preparations (pink dots and green squares, respectively; both from R. f. nippon ) caused by adduction of the thyroid over a distance up to ~500 μm towards the cricoid cartilage (ten trials each). Pink dots depict same preparation as shown in a and b , and horizontal dashed line indicates the fundamental of the resting frequency ( RF 1 =34.8 kHz) for this animal obtained in vivo . Ranges of echolocation (Echol. )pulses and communication calls for this subspecies indicated at right (same data as in Fig. 3f ). Full size image Figure 4b depicts average results of this switch to aperiodic sound emission from ten trials (same larynx preparation as in Fig. 4a ). It shows how frequency, bandwidth and amplitude changed with altering air pressure. Below approximately 2.1 kPa, increasing air pressures caused frequency changes similar to those depicted in Fig. 3 . Initially, the frequency ( Fig. 4b , blue dots in bottom panel) increased within F 1 high until a rapid downward shift to F 1 low around 1.9 kPa (red dots in Fig. 4b ). At approximately 2.1 kPa, the bandwidth of the signal suddenly increased ( Fig. 4b , pink squares in bottom panel). This marked the transition from periodic to aperiodic sound emission. Rapid transitions between periodic and aperiodic signals are also commonly found in naturally produced communication calls of horseshoe and other bats ( Fig. 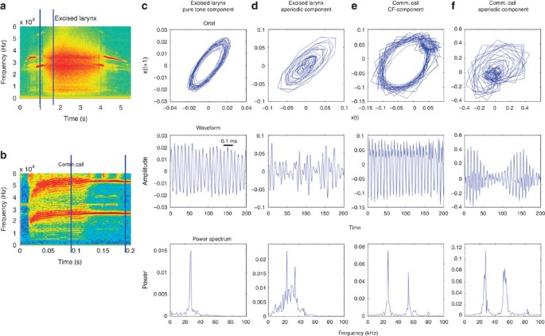4c ), accounting for almost 10% of a bat’s repertoire [4] , [21] . Figure 5: Features of periodic and aperiodic components in larynx phonations and natural communication calls. Sonagrams of a phonation of an excised larynx (a) and a natural communication (Commun.) call (b, similar toFig. 2c). (c–f) Spectral features analysed in a 0.8-ms time window at the time points indicated by vertical bars inaandb. Upper traces: embedded orbits of the extracted segment with a time delay of 0.004 ms. Centre traces: corresponding waveforms. Lower traces: corresponding power spectra. Figure 5 illustrates such spectro-temporal similarities between larynx phonations and natural horseshoe bat calls. Figure 5: Features of periodic and aperiodic components in larynx phonations and natural communication calls. Sonagrams of a phonation of an excised larynx ( a ) and a natural communication (Commun.) call ( b , similar to Fig. 2c ). ( c – f ) Spectral features analysed in a 0.8-ms time window at the time points indicated by vertical bars in a and b . Upper traces: embedded orbits of the extracted segment with a time delay of 0.004 ms. Centre traces: corresponding waveforms. Lower traces: corresponding power spectra. Full size image Simulated cricothyroid contractions The cricothyroid appears to be the sole laryngeal muscle controlling call frequencies in bats [5] , [6] . We examined its role in sound production by simulating its contractions. For this purpose, we adducted the thyroid cartilage towards the cricoid cartilage ( Fig. 3a ) over a total distance of up to 500 μm. This corresponded to a shortening of the cricothyroid by approximately 25–30%. As a result, the thyroid tilted downward, tautening the vocal folds ( Fig. 3a ). The subglottal air pressure remained unchanged and was set at a value that produced stable phonation of periodic signals within the range of F 1 high ( n =3) and F 1 low ( n =2), respectively. Figure 6a shows one representative trial for quasi-sinusoidal changes in adduction and the resulting variations in sound F 1 . When the cricothyroid cartilage was not adducted and presumably close to its resting position, call frequencies emitted at F 1 high were approximately 3.5 kHz below the bat’s RF 1 . Different degrees of adduction caused frequency changes that were highly linear for sounds emitted at both F 1 high and F 1 low . Figure 6c shows data for two preparations of R. f. nippon . We tested one preparation of R. f. tragatus for changes in F 1 high only and it also exhibited a linear correlation with R =0.86 (Pearson’s correlation, P <0.001, n >250). In the two cases depicted in Fig. 6c , adduction of the thyroid from 10 μm to over 400 μm increased the values for F 1 high from 30.5 to 34.8 kHz (regression line for pink dots; RF 1 of this bat was 33.8 kHz) and from 29.7 to 32.0 kHz (regression line for green squares). For the second harmonics, this corresponded to a range of 8.6 kHz (up to 6.6 kHz below and 2.0 kHz above the RF 2 of 67.6 kHz) and 4.6 kHz, respectively. This was sufficient to explain the range of natural echolocation pulses produced while at rest and during DSC [1] , [2] , [3] (note that sounds emitted at F 1 high for adductions of more than approximately 400 μm became extremely weak and virtually disappeared in the background noise; these data were therefore not included). For sound frequencies emitted at F 1 low , thyroid adductions yielded average frequencies that increased from 21.4 to 27.5 kHz (regression line for pink dots) and from 23.0 to 27.0 kHz (regression line for green squares). The average second harmonics for F 1 low therefore reached frequencies that were only 3.0 and 2.7 kHz, respectively, lower than the lowest values emitted for F 1 high . For the case in which we were able to determine RF 2 in vivo (pink dots), the second harmonics reached on an average up to 24.8 kHz below RF 2 , which matched the frequency difference observed between echolocation and most communication signals ( Fig. 1 ). The rates of frequency change per 100 μm movement of the thyroid cartilage were 0.6 and 1.2 kHz for F 1 high , and 0.6 and 1.1 kHz for F 1 low . In summary, combining the linear frequency changes of F 1 high and F 1 low that were caused by thyroid adductions at the two different air flows covered virtually the entire range of the call repertoire of horseshoe bats [4] ( Fig. 6c ). Our data show that changes in subglottal air pressure within a naturally occurring range [20] were sufficient to reproduce many features of natural vocalizations in horseshoe bats. Most notably, they were small linear frequency changes and non-linear jumps between frequency bands used for echolocation and communication, respectively. This indicates that these characteristics are based on biomechanical properties of the horseshoe bat larynx and do not require neuromuscular control by the brain. Many other vertebrate larynges exhibit similar frequency jumps, including in humans, where they reflect ‘register changes’ [16] , [22] , [23] , [24] , [25] , such as the switch from chest voice to falsetto during yodelling. Such register changes result from changes in vocal-fold vibrations. Therefore, only direct measurements of these vibrations will of course determine how they relate to acoustic features that one observes in larynx phonations. Nevertheless, what distinguishes the observations in horseshoe bats is that the frequency bands occupied by the two states matched the two major frequency bands that these bats use for sonar and social communication, respectively. It is therefore tempting to speculate that a behaviour similar to yodelling enables horseshoe bats to switch between echolocation and communication. Borrowing terminology used for the human voice, our bats would then emit communication sounds, for example, in ‘modal’ or ‘chest voice’, and echolocation pulses in ‘falsetto’. We measured the effects of changes in air pressure on sound production in excised larynges, similar to studies in humans [26] , [27] , dogs [28] or the bird syrinx [16] . Therefore, this raises the question how sound production may differ between in vitro and in vivo conditions. An excised larynx (or syrinx) may show a reduced structural stability and/or it may exhibit different air pressures [22] . We are aware of only one study that examined differences between in vitro and intact vocal organs, the zebra finch syrinx, in detail [29] . The authors found that non-linearities occurred only in vitro , probably because of altered air pressures. The sudden rapid acoustic transitions observed in natural zebra finch song are therefore most likely caused by direct control from superfast muscles [29] , [30] . Results from preparations of excised vocal organs therefore should always be interpreted cautiously. Nevertheless, pressures in the in vitro preparations of humans, dogs and our horseshoe bats, on the other hand, were similar to the natural pressures measured in vivo [20] , [26] , [27] , [28] . Although it is impossible to determine whether the anatomical position of the cartilages (and therefore of the muscles) in our in vitro preparations corresponded to the condition in vivo , we found numerous striking similarities between phonations produced by excised larynges and natural vocalizations; the frequency bands of F 1 high and F 1 low matched the frequency ranges of echolocation and communication calls. This even occurred in two subspecies with very different average frequencies of their echolocation and communication calls ( Fig. 3f ). In addition, the frequency ranges that we produced by simulating cricothyroid contractions corresponded extremely well with the ranges naturally used for echolocation (DSC) and communication ( Fig. 5c ). Finally, RFs measured in live bats just a few days before we examined their excised larynges also fell within the proper range of F 1 high frequencies produced by the excised larynx ( RF 1 in Figs 3c and 6c ). What causes linear frequency changes in horseshoe bat vocalizations? Although changes in air pressure did produce smooth, gradual changes of F 1 high and F 1 low , it seems unlikely that changes in air pressure alone are the immediate cause for linear call frequency changes in live bats: Echolocating and flying horseshoe bats can change the CF portion of their second harmonics during DSC between 6 kHz below and 1.5 kHz above their RF 2 [1] , [2] , [3] , and communication call frequencies vary by at least 10 kHz [4] . In comparison, subglottic pressure changes generated much smaller frequency changes (2.76±0.67 kHz for F 1 high and 3.25±0.81 kHz for F 1 low , that is, twice the amount for the second harmonics emitted by live bats). Variations in subglottic pressure alone are therefore insufficient to explain the entire range of echolocation and communication call frequencies produced by live bats. Other work also indicates that the subglottal pressure has only a limited, if any, effect on the frequency of bat echolocation pulses [31] . Instead, cricothyroid contractions most likely represent the major source for these linear changes, but only within each of the frequency bands. When we simulated cricothyroid contraction, the phonation frequencies changed linearly within the frequency bands of either F 1 high (echolocation) or F 1 low (communication). This limitation is most likely not caused by an insufficient adduction of the thyroid cartilage for several reasons. The amount of cricothyroid shortening that we simulated in our preparations corresponds to length changes observed in other larynx preparations [32] , [33] . It also represents the upper limit of adduction in human larynges [31] . Linear relationships between vocal pitch and the distance between cricoid and thyroid cartilage have also been reported in humans [34] . Similarly, electrical stimulations of the cricothyroid muscle in horseshoe bats revealed highly linear call frequency changes [5] , although the data were limited to the narrow range between RF 2 and 1.2 kHz above. Neurophysiological recordings from the cricothyroid muscle, its motor nerve, the superior laryngeal nerve and from neurons in the nucleus ambiguus demonstrated a linear decline in spike activity from about 40 to 10 spikes s −1 with decreasing call frequency from RF 2 to 3–5 kHz below [5] , [7] , [35] (see also Supplementary Fig. 1 ). Extrapolating these data suggests that the neuronal activity would cease only 5–6 kHz below RF 2 . Even if spike activities did not completely cease at these lower call frequencies, it is challenging to imagine how such extremely reduced spike levels could encode for the large modulations in call frequencies seen in communication calls ( Fig. 1 ). The frequency range covered by linear changes in spike activity corresponds only to the frequencies produced by simulated cricothyroid contractions at F 1 low ( Fig. 4c ). This covers the range of call frequencies emitted during echolocation, including DSC [1] , [2] , [3] , but not lower-pitched communication signals. Assuming that the cricothyroid is the sole, or at least the major, muscle responsible for call frequency control in bats [5] , [20] , horseshoe bats could generate all behaviourally relevant call frequencies, therefore, only by combining linear changes in frequency caused by cricothyroid contraction with non-linear effects from varying subglottal air pressure. In addition to direct tension control of the mammalian vocal fold by a single larynx muscle, such as the cricothyroid, however, other mechanisms may also affect vocal-fold tension and thus phonation frequency. For example, additional muscles, such as the thyroarytenoid [11] , [15] or changes in the subglottal pressure [12] , [14] , [36] could also contribute. Finally, when muscle contractions or relaxations approach their maxima, non-linear relationships between muscle contractions and the resulting vocal-fold tension may occur. Nevertheless, various evidence suggests that the cricothyroid represents the major source for call frequency control in bats. Only sections of the superior laryngeal, not of the recurrent nerve, lowered call frequency and amplitude [5] , [6] , [20] . Conversely, only spike activities of the superior laryngeal nerve correlated with call frequencies [7] , [37] . Finally, simulated contractions of the cricothyroid yielded phonation frequencies that strikingly matched the frequencies emitted during echolocation and communication, including RFs that we obtained from individual live bats. In conclusion, it appears therefore that the neural networks that control the activity of the cricothyroid muscle and those that generate the subglottal air pressure through the amount of adduction of the vocal folds are more tightly interconnected than previously assumed [38] , [39] . The cricothyroid is innervated by the superior laryngeal nerve, whose motoneurons are located in the anterior portion of the nucleus ambiguus [5] , [7] , [37] . In contrast, vocal-fold adduction is controlled by the recurrent laryngeal nerve, which originates from motoneurons in the posterior nucleus ambiguus [7] , [35] , [40] . Hence, we generally assumed that separate motor circuits mediate spectral and temporal call features, and supralaryngeal nerve activity would account for call frequency. On the other hand, the recurrent laryngeal nerve would control the amount of opening and closing of the glottis, that is, vocal-fold adduction and thus determine mostly the temporal call features [7] , [35] , [38] , [39] , [40] . The data presented here indicate, however, that call frequency changes involve more than merely supralaryngeal motor commands and contractions of the cricothyroid. They also require coordinating vocal-fold adduction with subtle modulations of the subglottal air flow. The latter result in non-linear changes in vocal-fold vibrations that give rise to sudden jumps in laryngeal phonations. Therefore, the neural circuit that controls glottal air flow not only determines temporal features, such as on- and offset and the amplitude of calls, but also allows bats to switch between generating echolocation and communication calls. In addition, it is intricately linked with neuromuscular control of the cricothyroid. Call amplitudes are also intricately linked with contractions of expiratory, mostly abdominal muscles [41] , which are innervated by spinal nerves. How these different motoneuron pools achieve such a precise gating of activity is currently unknown. Finally, it is important to note that recent phylogenetic evidence suggests that several acoustic features of bat echolocation evolved convergently multiple times, and horseshoe bats with their sophisticated echolocation share a common ancestry with non-echolocating old-world fruit bats [42] . This implies that there is most likely more than one design principle for the neural circuits and mechanisms underlying bat echolocation. Animals Greater horseshoe bats, Rhinolophus ferrumequinum , were collected in China and belonged to two different subspecies with slightly different call features (see Results): three males and three females (from Beijing) belonged to R. f. tragatus , and two males and three females belonged to R. f. nippon (from Ji An/Jilin). Procedures were in accordance with National Institute of Health guidelines for experiments involving vertebrate animals and were approved by University of California, Los Angeles’ Institutional Animal Care and Use Committee. Preparation and setup Following the approach of Fee et al . [16] for the bird syrinx, we removed larynx, trachea and both lung lobes from the bat, cleaned them of excess connective tissue and mounted them on the experimental platform. We cut the vocal tract immediately dorsal to the epiglottis ( Fig. 3b ; length of attached trachea between larynx and bronchial branches, approximately 13 mm) and inserted a small piece of polyethylene tubing (2 cm long, inner diameter 1.14 mm, outer diameter 1.57 mm; Clay Adams Inc., New York, NY, USA) into the trachea and held it in place with a string. The opposite end of the tubing was inserted into a polyvinyl chloride tubing (inner diameter 4.7 mm, outer diameter 7.9 mm; Fisher Scientific, Pittsburg, PA, USA) and connected to a jar providing warm, humid air (temperature: 35–40 °C; humidity: >94%) via a pressurized air outlet with manually adjustable pressure. We measured subglottal changes in air pressure with an electric pressure sensor (MPX5050DP; Freescale Semiconductor, Austin, TX, USA), which was inserted into the tubing close to the trachea. We determined absolute tracheal air pressures based on the pressure measured by the sensor and corrected for the 0.45 times smaller diameter of the tubing inserted into the trachea. We varied tracheal air pressures over a range of approximately 3.5 kPa. Applying isotonic saline solution (0.9% NaCl) to the surface of the larynx and trachea every 5 min maintained a moist preparation during experimental procedures. To simulate contraction of the cricothyroid muscle, we altered the distance between the thyroid and cricoid cartilage with a pair of forceps (Dumont #5; Fine Science Tools, Foster City, CA, USA; width of tips: approximately 50 μm) and an attached slide potentiometer (linear motion, Type V448 MONO, CTS Electronic Components, Kaohsiung, Taiwan). This allowed us to quantify the simulated cricothyroid motion with an accuracy of 15 μm (standard error of potentiometer). Experimental procedure Before we began to systematically measure the effects of varying air flow on sound production, we determined the overall range of air pressure that generated sound. For this purpose, we increased air pressure linearly from a level slightly below the lowest level at which sounds were produced and then decreased it again. Subsequently, we varied air pressure over this range at least ten times for a period of 1–5 s each. We simulated cricothyroid muscle contractions by changing the distance between the cricoid and thyroid cartilage with a pair of forceps. One tip of the measuring forceps was placed immediately above the protruding rostroventral edge of the thyroid and the other tip immediately below the equally bulging caudoventral edge of the cricoid cartilage (see Fig. 2a ). We used a resistor positioned between the shanks of the forceps to measure the changes in the distance between the tips by converting them into changes in DC voltage. Particular care was taken not to damage the laryngeal tissue and, therefore, the forceps were not permanently attached to the cartilages (for example, by glueing them to the tissue) but merely touched the edges of the cartilages. Therefore, we could only compress the forceps simulating muscle contraction. Relaxation of the cricothyroid muscle could not be measured reliably and was therefore not analysed. Recording procedure, data analysis and statistical analysis We used a 1/4 ultrasonic microphone (4,939 with pre-amplifier 2633, Brüel & Kjær, Nærum, Denmark), positioned at a distance of 15 cm from the rostral end of the larynx to record the phonations. The recording system had a flat frequency response of ±3 dB between 10 and 100 kHz. Sound signals and outputs of the pressure sensor and the resistor were recorded (16 bit, 300 kHz sample rate; UltraSoundgate 116, Avisoft Bioacoustics, Berlin, Germany) and analysed with commercial analysis software (SASLab Pro; Avisoft Bioacoustics; length of fast Fourier transformation (FFT): 1,024 points with 94% overlap, spectral resolution: 195 Hz). We determined the bandwidth of aperiodic signals by measuring the width of the power spectrum 30 dB below the peak. Statistical analysis was performed using the Pearson’s correlation coefficient (level of significance: probability of error <5%). How to cite this article: Kobayasi, K. I. et al . Behavioural and neurobiological implications of linear and non-linear features in larynx phonations of horseshoe bats. Nat. Commun. 3:1184 doi: 10.1038/ncomms2165 (2012).